Systemic control of immune cell development by integrated carbon dioxide and hypoxia chemosensation inDrosophila Drosophila hemocytes are akin to mammalian myeloid blood cells that function in stress and innate immune-related responses. A multi-potent progenitor population responds to local signals and to systemic stress by expanding the number of functional blood cells. Here we show mechanisms that demonstrate an integration of environmental carbon dioxide (CO 2 ) and oxygen (O 2 ) inputs that initiate a cascade of signaling events, involving multiple organs, as a stress response when the levels of these two important respiratory gases fall below a threshold. The CO 2 and hypoxia-sensing neurons interact at the synaptic level in the brain sending a systemic signal via the fat body to modulate differentiation of a specific class of immune cells. Our findings establish a link between environmental gas sensation and myeloid cell development in Drosophila . A similar relationship exists in humans, but the underlying mechanisms remain to be established. Carbon dioxide (CO 2 ) is the first identified gaseous molecule that evokes innate avoidance behavior in Drosophila [1] , and is a critical sensory and respiratory cue that alters a variety of animal behaviors [2] . CO 2 is detected by a heterodimeric receptor encoded by Gr21a and Gr63a that is expressed in the terminal organ of the larval head or in the antennal olfactory receptor neurons called ab1C in adult flies [3] , [4] . Even though CO 2 was initially identified as a stress molecule, fruits, yeast, and animals emit CO 2 as a respiration by-product that lead to complex combinatorial responses to odorants [5] . Drosophila hemocytes are akin to mammalian myeloid cells and are sentinels for stress and innate immune-related responses [6] , [7] . Drosophila hemocytes arise from multi-potent blood progenitors and are comprised of three representative classes of myeloid-like cells: plasmatocytes, crystal cells (CCs), and lamellocytes [8] . The majority of mature hemocytes are macrophage-like plasmatocytes while a small fraction becomes CCs known to function in wound healing and innate immune responses [7] , [9] . Lamellocytes are seldom found in conventional culture conditions and are evident only upon immune challenge [10] . The maintenance of hematopoietic stem- and progenitor populations and their interactions with the niche has been extensively studied in both humans and in model systems [6] , [8] , [11] , [12] . However, the importance of extrinsic cues that originate outside the stem- or progenitor compartment has not been carefully characterized and requires extensive future studies. Complex systemic responses often involve multiple organs and a combination of developmental and stress-related signals [13] . With the use of modern genetic techniques, the Drosophila hematopoietic system allows us to delineate mechanistic insights into intricate responses of the myeloid progenitor population to multiple systemic signals [14] , [15] , [16] . However, how sensory neurons that detect the level of ambient gases communicate with the myeloid blood system has not been elucidated although functional analogies have been identified in mammals. In this study, we identify a genetic link between the respiratory gas-chemosensation and myeloid blood development in Drosophila . CO 2 -sensing and hypoxia-sensing neurons interact at the synaptic level. Low CO 2 or O 2 triggers the stabilization of Hypoxia inducible factor-α in a small set of neurons in the ventral nerve cord (VNC), promoting transcription of the cytokine unpaired3 in the brain. This secreted cytokine activates the JAK/STAT pathway in fat bodies (considered similar to the liver), resulting in the expression and secretion of an insulin-like protein, Dilp6. This secreted protein activates the insulin receptor in the hematopoietic organ and this leads to increased levels of the protein Serrate, a ligand for Notch. Increased Notch signaling raises the number of a specific class of immune cells. Notably, this phenotype is recapitulated by modulating atmospheric CO 2 or O 2 , emphasizing that gas perception is directly associated with differentiation of the hematopoietic system in Drosophila . Respiratory chemosensation and CC differentiation CO 2 activates a transmembrane, heterodimeric gustatory receptor complex, called Gr21a/Gr63a [3] , [4] . It is specifically expressed in the terminal organ of the larval head (Supplementary Fig. 1a ). Other tissues, including the hematopoietic organ called the lymph gland (Fig. 1a ), do not express this receptor (Supplementary Fig. 1b ). The CO 2 -sensing neuron (CO 2 SN for simplicity) sends its projection to the subesophageal ganglion (SEG), which in turn connects, through largely unmapped circuits, to the central brain and VNC [3] , [4] , [17] . Receptors capable of responding to oxygen levels (or monoxide gases and free radicals) are more widely expressed and belong to the intracellular soluble guanylyl cyclase class of proteins [18] , [19] . The receptor Gyc89da is activated by low molecular oxygen (O 2 ) and the multiple neurons expressing it specifically sense hypoxia (HypSNs for simplicity). HypSNs are inhibited in normoxia and hyperoxia [20] , [21] . Fig. 1 CO 2 chemosensation controls the differentiation of crystal cells. Graphs indicate the number of crystal cells (CC) per lymph gland lobe. Bars in graphs: the median. n.s: not significant ( p > 0.01). * p < 0.01; ** p < 0.001; *** p < 0.0001. Scale Bar: 20μm. White dotted lines: lymph glands. Statistical results and genotypes are indicated in Supplementary Table 3 . a A schematic representation of the primary lobe of the hematopoietic organ, the larval lymph gland. 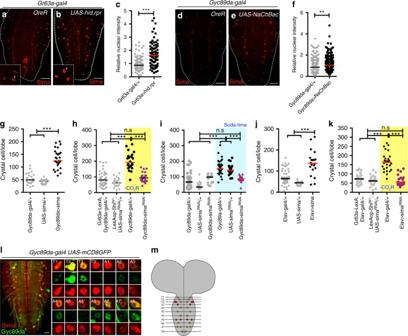Fig. 3 Sima (Hifα) stabilization in HypSNs affects crystal cell number.candfindicate the relative intensities of nuclear Sima, and Graphs ing–kindicate the number of CCs in a single lymph gland lobe. n.s: not significant (p> 0.01). *p< 0.01; **p< 0.001; ***p< 0.0001. Scale Bar: 50μm. Bars in graphs: the median. CO2SN inhibited conditions: –CO2R with shaded yellow inh, k, and Soda-lime generated low CO2: shaded blue inifor clarity.a–cInhibition of the CO2SN elevates Sima expression in the VNC. Control brains (Gr63a-gal4/+) exhibit very low Sima expression in the VNC (Sima is in red) (a). Genetic ablation of CO2SN (Gr63a-gal4; UAS-hid,rpr) leads to 2-fold increase in accumulation of nuclear Sima in specific VNC cells (white arrows in inset) (b). Quantitation of data shown inc.d–iActivation of HypSNs elevates Sima expression in the VNC. Control brains (Gyc89da-gal4/+) show very low Sima expression (d). Constitutive activation of HypSNs significantly increases accumulation of nuclear Sima in specific VNC cells (Gyc89da-gal4; UAS-NaChBac) (e). Quantitation of relative nuclear Sima intensity shown inf. CC differentiation is significantly enhanced whensimais overexpressed in HypSN cells (Gyc89da-gal4; UAS-sima) (g).simaRNAiexpressed in HypSNs suppresses the extra CC differentiation phenotype caused by loss of CO2SN function (Gr63a-LexA, LexAop-Shits1; Gyc89da-gal4, UAS-simaRNAi) (h). This rescue is also seen upon loss ofsimain HypSNs when animals are grown in low CO2(soda-lime) condition (i).j-ksimaexpression in neurons is linked to CC differentiation. Larvae expressingsimain the brain (Elav-gal4; UAS-sima) facilitates CC differentiation (j). Also, increased CC differentiation caused by CO2SN inhibition is rescued by concurrent inhibition ofsimain the brain (Gr63a-LexA, LexAop-Shits1; Elav-gal4, UAS-simaRNAi) (k).l,mSima co-localizes with a subset of HypSNs. Within the VNC, neurons express Sima in total 14 pairs per hemineuromere from T1 to A8. Amongst these, 10 pairs co-localize with Gyc89da in the T1-T3, A2-A4 and A6-A8 (Gyc89da-gal4; UAS-mCD8GFP). A magnified view of Sima and Gyc89da-expressing neurons in the thoracic and abdominal ganglia (Sima, red; Gyc89da, green) (l). In the reconstructed image of VNC, Sima+HypSNs are shown in yellow and Sima+cells that are not HypSNs are marked in red (m) Undifferentiated blood progenitors reside in the inner core, termed the medullary zone (MZ), and give rise to mature blood cell lineages including crystal cells (CC, marked in yellow) that occupy a region termed the cortical zone (CZ). The posterior signaling center (PSC) secretes multiple factors to maintain the progenitors. Only the features relevant to this study are shown. b–l Loss of CO 2 SN activity causes increased CC number. Wild-type third-instar larvae express fewer than 100-CCs per primary lymph gland lobe (CCs are marked in red, Lz) ( b ) Both homozygous ( Gr63a 1 / Gr63a 1 ) ( c ) and heterozygous ( Gr63a 1 /+) mutants ( d ) of Gr63a , the gene encoding the chemoreceptor for CO 2 sensing, exhibit increased numbers of CCs. Quantitation of CC numbers shown in ( e ). Gr21a encodes the second subunit of the CO 2 chemoreceptor that functions with Gr63a . Knockdown of Gr21a function ( Gr63a-gal4; UAS-Gr21a RNAi ) ( f ), or genetic ablation of the CO 2 receptor neuron by expression of pro-apoptotic genes, hid and rpr ( Gr63a-gal4; UAS-hid,rpr ) ( g ) or attenuation of synaptic transmission by expression of a temperature-sensitive form of the dynamin-like protein Shibire ( Gr63a-gal4; UAS-Shi ts1 ) ( h ), each causes a significant increase in the number of CCs. This phenotype is not observed in Gal4 - or UAS -controls alone. Quantitation is shown in i . Absorption of ambient CO 2 in larval culture vial with the use of soda-lime, a mixture of bases that eliminates gaseous CO 2 (see Methods for detail), mimics the CO 2 SN mutant phenotype ( j ). This phenotype is enhanced by a simultaneous knockdown of Gr21a in the CO 2 SN ( Gr63a-gal4; UAS-Gr21a RNAi ) ( k ). Quantitation shown in l . The blue shading in panels ( l ) represents soda-lime-induced low environmental CO 2 condition Full size image We modified the activities of the CO 2 SN or the HypSNs using a variety of genetic and environmental manipulations (Supplementary Fig. 1c ). As a hematopoietic readout, we count CCs, which function in wound healing, clotting, innate immunity, and hypoxic stress response [9] , [22] , [23] . Compared with wild-type larvae raised under conventional environmental conditions, we find between 2 and 4-fold increase in the number of CCs upon reduced CO 2 SN activity (Fig. 1 b-l and Supplementary Fig. 1 d-l). This phenotype is specific to the CCs and does not alter the number of other cell types or the overall size of the lymph gland (Supplementary Fig. 1 m-o). Also, the numbers of sessile and circulating CCs within the larvae are not affected (Supplementary Fig. 1 p-s). Loss of HypSN activity has no effect on CC number (Fig. 2a, b, d ) while elevated activity of HypSNs causes 2-fold increase in CCs (Fig. 2c, d ) when specifically activated in neurons (Fig. 2e–g and Supplementary Fig. 1t ). This phenotype is recapitulated upon inhibition of neuronal Gyc89da (Supplementary Fig. 1u ). Thus, low CO 2 SN activity (low CO 2 availability) or high HypSNs activity (low O 2 availability) favors extra CC formation. Fig. 2 CO 2 SN forms inhibitory synapses with HypSN. Graphs indicate the number of crystal cells (CC) per lymph gland lobe. Bars in graphs: the median. n.s: not significant ( p > 0.01). * p < 0.01; ** p < 0.001; *** p < 0.0001. Scale Bar: 20μm, unless otherwise indicated. White dotted lines: lymph glands. CO 2 SN inhibited conditions: –CO 2 R with shaded yellow in i , and Soda-lime generated low CO 2 : shaded blue in k for clarity. a–g Constitutive activation of HypSNs induces CC differentiation. Control animals ( Gyc89da-gal4/ + ) have an average of 70-90 CCs ( a ). Inactivation of HypSNs ( Gyc89da-gal4; UAS-Shi ts1 ) does not alter CC number ( b ). Constitutive activation of HypSNs by expressing the bacterial sodium channel, NaChBac ( Gyc89da-gal4; UAS-NaChBac ) results in increased CC differentiation ( c ). Quantitation is shown in d . When the expression of NaChBac is specifically blocked in neurons ( Gyc89da-gal4, Elav-gal80; UAS-NaChBac ) the average CC number is unchanged ( f ) from that in control ( e ). Quantitation shown in g . h–k HypSNs function downstream of CO 2 SN. As shown in (Fig. 1h ), CO 2 SN inhibition increases CC number ( Gr63a-gal4; UAS-Shi ts1 ). This phenotype reverts to wild type when HypSNs are also inhibited ( Gr63a-gal4; Gyc89da-gal4, UAS-Shi ts1 ) ( h ). Quantitation shown in i . Soda-lime-mediated CC phenotype is also alleviated by inhibition of HypSNs (low atmospheric CO 2 + Gyc89da-gal4; UAS-Shi ts1 ) ( j ). Quantitation shown in k . l–m GABA-mediated inhibition of HypSNs by CO 2 SN. Knockdown of Gad1 in the CO 2 SN ( Gr63a-gal4; UAS-Gad1 RNAi ) enhances differentiation of CCs ( l ). Similarly, loss of either GABA B R1 or GABA B R2 in HypSNs ( Gyc89da-gal4; UAS-GABA B R1 RNAi or Gyc89da-gal4; UAS-GABA B R2 RNAi ) also leads to increased CC differentiation ( m ). n–o Physical proximity and overlap of CO 2 SN and HypSNs in the SEG. Projections of the CO 2 SN adjoining HypSNs at the level of the SEG shows significant co-localization: CO 2 SN in red and HypSN in green ( Gr63a-gal4; UAS-DenMark; Gyc89da-GFP ). Rendered image of the co-localization data shown in right panel ( n ). Syb::GRASP expression of the CO 2 SN and HypSNs in the SEG ( o ). Syb::GRASP signal resulting from points of contact is shown in green (Magnified images in the following panels) ( o ) . p Negative control experiments for the Syb::GRASP data shown in o . Gr63a-LexA alone ( Gr63a-LexA; UAS-CD4-spGFP 11 , LexAop-nSyb-spGFP 1-10 ) or Gyc89da-gal4 alone ( Gyc89da-gal4; UAS-CD4-spGFP 11 , LexAop-nSyb-spGFP 1-10 ) does not give rise to a GRASP signal. Scale bar: 50μm Full size image The increased CC phenotype due to low CO 2 SN activity is fully suppressed to wild-type numbers by concurrent low HypSN activity (Fig. 2h–k ), raising the possibility of a coupled response. An RNA i -based mini-screen for enzymes that synthesize neurotransmitters revealed that knockdown of Gad1 (encoding the GABA synthesis enzyme, glutamate decarboxylase) in the CO 2 SN gives increased CC numbers (Fig. 2l and Supplementary Fig. 1v ). Remarkably, knockdown of the GABA B receptors, R1/R2 in the HypSNs similarly raises CC numbers (Fig. 2m and Supplementary Fig. 1w, x ). This prompted us to investigate a possible direct interaction between these neurons at inhibitory synapses. We expressed the dendritic marker, DenMark [24] , in the CO 2 SN and simultaneously marked HypSNs with GFP. Separate neurons with nuclei residing within the terminal ganglion express these two receptors. Although both send anterior projections to the terminal organ, at this location, they appear to be non-overlapping (Supplementary Fig. 1y ). In contrast, the posterior projection from the single CO 2 SN approaches the SEG, where it comes into extremely close association with a projection from HypSNs (Fig. 2n ). We next utilized the GRASP technique [25] , [26] , in which a positive fluorescence signal indicates molecular level proximity between the two neurons. Using membrane-GRASP, we detect such close association between the CO 2 SN and the HypSNs at the level of the SEG (Supplementary Fig. 1z , aa). For even finer analysis, we used Synaptobrevin::GRASP that would only highlight points of active synaptic contacts (Full genotype: Gyc89da-gal4; Gr63a-LexA, UAS-CD4-spGFP 11 , LexAop-nSyb-spGFP 1-10 ). Punctate signals are readily evident in the anterior SEG indicating synapse formation between these two classes of neurons (Fig. 2o, p ). Taken together, the genetic data on the involvement of GABAergic neurons, the DenMark data on proximity of labeled branches and the GRASP analyses, we conclude that the CO 2 SN forms inhibitory synapses with HypSN branches at the level of the SEG. These data do not preclude additional parallel interactions elsewhere within the neuronal circuitry of the central brain. Attenuation of CO 2 SN stabilizes Hifα in HypSNs in the VNC Hypoxic conditions allow stabilization of Hypoxia inducible factor-α (Hifα, called Sima in Drosophila ) and favor CC differentiation through non-canonical activation of Notch [27] . A small number of cells in the VNC express very low levels of Sima protein even in wild-type larvae grown under normoxic conditions (Fig. 3a ) and this Sima protein expression is upregulated if CO 2 SN activity is attenuated (Fig. 3b, c ), or if HypSN activity is increased (Fig. 3d–f ). Additionally, loss of Gad1 in the CO 2 SN raises Sima levels in the VNC neurons (Supplementary Fig. 2 a-c), highlighting the interaction between CO 2 SN and HypSNs in this process. Overexpression of sima in HypSNs is sufficient to induce increased CC differentiation under normal gaseous ligand sensation (Fig. 3g and Supplementary Fig. 2d ). Also, knockdown of sima transcript in HypSNs rescues the CC phenotype seen under low CO 2 SN activity (Fig. 3h, i and Supplementary Fig. 2 e-g). These two results are also seen if sima levels are manipulated specifically in all neurons (Fig. 3j, k and Supplementary Fig. 2 g-i). Thus, no non-neuronal participant is essential and Sima increase in HypSNs is both necessary and sufficient for linking the sensory signals to CC formation. The high VNC Sima expression is seen in 14 pairs of neurons of which 10 pairs are HypSNs (Fig. 3l, m ). These results establish that HypSNs that are also Sima + are important for the CC phenotype. Fig. 3 Sima (Hifα) stabilization in HypSNs affects crystal cell number. c and f indicate the relative intensities of nuclear Sima, and Graphs in g–k indicate the number of CCs in a single lymph gland lobe. n.s: not significant ( p > 0.01). * p < 0.01; ** p < 0.001; *** p < 0.0001. Scale Bar: 50μm. Bars in graphs: the median. CO 2 SN inhibited conditions: –CO 2 R with shaded yellow in h, k , and Soda-lime generated low CO 2 : shaded blue in i for clarity. a–c Inhibition of the CO 2 SN elevates Sima expression in the VNC. Control brains ( Gr63a-gal4/ + ) exhibit very low Sima expression in the VNC (Sima is in red) ( a ). Genetic ablation of CO 2 SN ( Gr63a-gal4; UAS-hid,rpr ) leads to 2-fold increase in accumulation of nuclear Sima in specific VNC cells (white arrows in inset) ( b ). Quantitation of data shown in c . d–i Activation of HypSNs elevates Sima expression in the VNC. Control brains ( Gyc89da-gal4/ + ) show very low Sima expression ( d ). Constitutive activation of HypSNs significantly increases accumulation of nuclear Sima in specific VNC cells ( Gyc89da-gal4; UAS-NaChBac ) ( e ). Quantitation of relative nuclear Sima intensity shown in f . CC differentiation is significantly enhanced when sima is overexpressed in HypSN cells ( Gyc89da-gal4; UAS-sima ) ( g ). sima RNAi expressed in HypSNs suppresses the extra CC differentiation phenotype caused by loss of CO 2 SN function ( Gr63a-LexA, LexAop-Shi ts1 ; Gyc89da-gal4, UAS-sima RNAi ) ( h ). This rescue is also seen upon loss of sima in HypSNs when animals are grown in low CO 2 (soda-lime) condition ( i ). j - k sima expression in neurons is linked to CC differentiation. Larvae expressing sima in the brain ( Elav-gal4; UAS-sima ) facilitates CC differentiation ( j ). Also, increased CC differentiation caused by CO 2 SN inhibition is rescued by concurrent inhibition of sima in the brain ( Gr63a-LexA, LexAop-Shi ts1 ; Elav-gal4, UAS-sima RNAi ) ( k ). l , m Sima co-localizes with a subset of HypSNs. 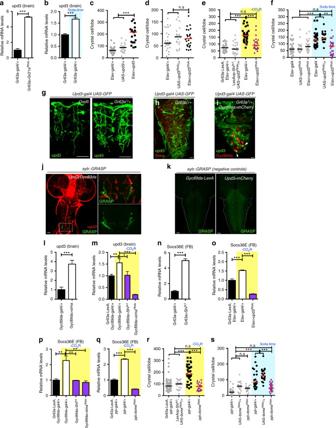Fig. 4 Upd3 secreted from the brain triggers a systemic signal.c–f,r–sindicate CC numbers in a single lymph gland. n.s: not significant (p> 0.01). *p< 0.01; **p< 0.001; ***p< 0.0001. Error bars ina–b,l–q: standard deviation. Bars inc–f,r–s: the median. Scale Bar: 50μm. CO2SN inhibited conditions: –CO2R with shaded yellow ine, m, o–r. Soda-lime generated low CO2conditions: shaded blue inb, f, s.a-bupd3upregulation in the brain is linked to CC differentiation. Loss ofGr21a(Gr63a-gal4;UAS-Gr21aRNAi) in the CO2SN (a) or scavenging of CO2(b) results in increasedupd3mRNA in the brain.c-m. Upd3 functions downstream of Sima.upd3in the brain causes increased CC formation (Elav-gal4; UAS-upd3) (c). Loss of neuronalupd3(Elav-gal4; UAS-upd3RNAi) alone does not alter CC number (d). Silencing neuronalupd3suppresses the CC phenotype caused by inhibition of CO2SN (Gr63a-LexA, LexAop-Shits1; Elav-gal4, UAS-upd3RNAi) (e) or by soda-lime treatment (Elav-gal4; UAS-upd3RNAi) (f). Compared with control,upd3is elevated in the posterior VNC ofGr63a1/ +mutants (Upd3-gal4, UAS-GFP; Gr63a1/ +) (g). No overlap is observed between Sima+andupd3+neurons (h). HypSN seen in the posterior VNC are occasionallyupd3-positive (white arrow heads), but the majority ofupd3+cells are not HypSNs (Upd3-gal4, UAS-GFP; Gyc89da-LexA; LexAop-mCherry) (i). Syb::GRASP expression of the HypSNs and Upd3+neurons in the VNC (Magnified images in the following panels) (Upd3, red; GRASP, green) (j).Gyc89da-LexAalone (Gyc89da-LexA; UAS-CD4-spGFP11, LexAop-nSyb-spGFP1-10) orUpd3-gal4alone (Upd3-gal4 UAS-mCherry; UAS-CD4-spGFP11, LexAop-nSyb-spGFP1-10) does not give rise to a GRASP signal (k). Overexpression ofsimain HypSNs increases neuronalupd3mRNA (Gyc89da-gal4; UAS-sima) (l).simaRNAior inhibition of HypSNs suppresses the elevatedupd3levels (Gr63a-LexA, LexAop-Shits1; Gyc89da-gal4, UAS-simaRNAior Gr63a-LexA, LexAop-Shits1; Gyc89da-gal4, UAS-Shits1) (m).n–sBrain-secreted Upd3 functions in the fat body.Socs36eis induced in the fat body upon loss of CO2SN (Gr63a-LexA; LexAop-Shits1) (n). This expression is suppressed upon: loss of neuronalupd3(Gr63a-LexA, LexAop-Shits1;Elav-gal4, UAS-upd3RNAi) (o), by simultaneous inhibition of HypSNs (Gr63a-LexA, LexAop-Shits1;Gyc89da-gal4, UAS-Shits1) (p), bysimaRNAiin the HypSNs (Gr63a-LexA, LexAop-Shits1;Gyc89da-gal4, UAS-simaRNAi) (p), or upon loss ofdomein the fat body (Gr63a-LexA, LexAop-Shits1;ppl-gal4, UAS-domeRNAi) (q).domeRNAiin the fat body reverts the CC numbers in the CO2SN mutant (Gr63a-LexA, LexAop-Shits1; ppl-gal4, UAS-domeRNAi) (r) or in soda-lime conditions (ppl-gal4; UAS-domeRNAi) (s) to wild-type Within the VNC, neurons express Sima in total 14 pairs per hemineuromere from T1 to A8. Amongst these, 10 pairs co-localize with Gyc89da in the T1-T3, A2-A4 and A6-A8 ( Gyc89da-gal4; UAS-mCD8GFP ). A magnified view of Sima and Gyc89da-expressing neurons in the thoracic and abdominal ganglia (Sima, red; Gyc89da, green) ( l ). In the reconstructed image of VNC, Sima + HypSNs are shown in yellow and Sima + cells that are not HypSNs are marked in red ( m ) Full size image Upd3 from the brain signals to the fat body VNC neurons are known to secrete hormones and cytokines into the hemolymph [28] . We conducted a targeted mini-screen of known hormone and secreted factor-encoding genes (Supplementary Fig. 3a ) to determine if any of these is differentially expressed at the mRNA level in the Gr63a mutant brain compared with controls. Three of these genes are upregulated in the mutant at the transcriptional level, of which only one, that encodes the cytokine unpaired3 ( upd3 ) gives increased CC numbers upon pan-neuronal overexpression (Fig. 4a–c and Supplementary Fig. 3b ). Loss of upd3 in neurons does not cause any hematopoietic defect (Fig. 4d ) but upd3-RNAi or upd3 mutants suppress the extra CC phenotype of CO 2 SN inhibition (Fig. 4e, f and Supplementary Fig. 3 c-f). This indicates a role for Upd3 in transmitting the gaseous ligand-generated stress signal to regions outside the brain. Fig. 4 Upd3 secreted from the brain triggers a systemic signal. c–f , r–s indicate CC numbers in a single lymph gland. n.s: not significant ( p > 0.01). * p < 0.01; ** p < 0.001; *** p < 0.0001. Error bars in a – b , l – q : standard deviation. Bars in c – f , r – s : the median. Scale Bar: 50μm. CO 2 SN inhibited conditions: –CO 2 R with shaded yellow in e, m, o–r . Soda-lime generated low CO 2 conditions: shaded blue in b, f, s . a-b upd3 upregulation in the brain is linked to CC differentiation. Loss of Gr21a ( Gr63a-gal4 ; UAS-Gr21a RNAi ) in the CO 2 SN ( a ) or scavenging of CO 2 ( b ) results in increased upd3 mRNA in the brain. c-m . Upd3 functions downstream of Sima. upd3 in the brain causes increased CC formation ( Elav-gal4; UAS-upd3 ) ( c ). Loss of neuronal upd3 ( Elav-gal4; UAS-upd3 RNAi ) alone does not alter CC number ( d ). Silencing neuronal upd3 suppresses the CC phenotype caused by inhibition of CO 2 SN ( Gr63a-LexA, LexAop-Shi ts1 ; Elav-gal4, UAS-upd3 RNAi ) ( e ) or by soda-lime treatment ( Elav-gal4; UAS-upd3 RNAi ) ( f ). Compared with control, upd3 is elevated in the posterior VNC of Gr63a 1 / + mutants ( Upd3-gal4, UAS-GFP; Gr63a 1 / + ) ( g ). No overlap is observed between Sima + and upd3 + neurons ( h ). HypSN seen in the posterior VNC are occasionally upd3 -positive (white arrow heads), but the majority of upd3 + cells are not HypSNs ( Upd3-gal4, UAS-GFP; Gyc89da-LexA; LexAop-mCherry ) ( i ). Syb::GRASP expression of the HypSNs and Upd3 + neurons in the VNC (Magnified images in the following panels) (Upd3, red; GRASP, green) ( j ). Gyc89da-LexA alone ( Gyc89da-LexA; UAS-CD4-spGFP 11 , LexAop-nSyb-spGFP 1-10 ) or Upd3-gal4 alone ( Upd3-gal4 UAS-mCherry; UAS-CD4-spGFP 11 , LexAop-nSyb-spGFP 1-10 ) does not give rise to a GRASP signal ( k ). Overexpression of sima in HypSNs increases neuronal upd3 mRNA ( Gyc89da-gal4; UAS-sima ) ( l ). sima RNA i or inhibition of HypSNs suppresses the elevated upd3 levels ( Gr63a-LexA, LexAop-Shi ts1 ; Gyc89da-gal4, UAS-sima RNAi or Gr63a-LexA, LexAop-Shi ts1 ; Gyc89da-gal4, UAS-Shi ts1 ) ( m ). n–s Brain-secreted Upd3 functions in the fat body. Socs36e is induced in the fat body upon loss of CO 2 SN ( Gr63a-LexA; LexAop-Shi ts1 ) ( n ). This expression is suppressed upon: loss of neuronal upd3 ( Gr63a-LexA, LexAop-Shi ts1 ; Elav-gal4, UAS-upd3 RNAi ) ( o ), by simultaneous inhibition of HypSNs ( Gr63a-LexA, LexAop-Shi ts1 ; Gyc89da-gal4, UAS-Shi ts1 ) ( p ), by sima RNA i in the HypSNs ( Gr63a-LexA, LexAop-Shi ts1 ; Gyc89da-gal4, UAS-sima RNAi ) ( p ), or upon loss of dome in the fat body ( Gr63a-LexA, LexAop-Shi ts1 ; ppl-gal4, UAS-dome RNAi ) ( q ). dome RNA i in the fat body reverts the CC numbers in the CO 2 SN mutant ( Gr63a-LexA, LexAop-Shi ts1 ; ppl-gal4, UAS-dome RNAi ) ( r ) or in soda-lime conditions ( ppl-gal4; UAS-dome RNAi ) ( s ) to wild-type Full size image Under conditions of reduced CO 2 SN activity, upd3 is detected in a large number of cells in the brain that are not obligatorily HypSNs or Sima + (Fig. 4 g, h). Yet, upd3 and HypSNs co-localize and synapse onto each other at the posterior region of VNC (Full genotype: Upd3-gal4, UAS-mCherry; Gyc89da-LexA, UAS-CD4-spGFP 11 , LexAop-nSyb-spGFP 1-10 ) (Fig. 4i–k ). Consistently, experimental evidence presented below suggests that the observed increase in upd3 is critically dependent on Sima + HypSNs. Overexpression of sima in HypSNs is sufficient to induce a 4-fold increase in upd3 transcription in the brain (Fig. 4l ). Also, loss of sima in HypSNs rescues the high upd3 transcription in a reduced CO 2 SN activity background (Fig. 4m ). Simultaneous loss of CO 2 SN and HypSN activities gives wild-type levels of upd3 transcription (Fig. 4m ). Socs36e is a direct downstream transcriptional target of the JAK/STAT signaling pathway initiated by Upd3 upon binding its receptor, Domeless (Dome) [29] . qPCR analysis of dissected tissues from larvae lacking CO 2 SN activity shows upregulation of Socs36e specifically in the fat body (considered similar to the liver) (Fig. 4n ), and importantly, not in the lymph gland (Supplementary Fig. 3g ). Fat body Socs36e expression is suppressed when either: upd3 is down-regulated in the brain, or when sima expression is decreased within HypSNs, or upon simultaneous inhibition of CO 2 SN and HypSNs (Fig. 4o, p ). Additionally, overexpression of either sima or upd3 in the brain is sufficient to induce Socs36e in the fat body (Supplementary Fig. 3h, i ). Finally, dome - RNAi autonomously suppresses Socs36e in the fat body and non-autonomously affects CC number in CO 2 SN activity-depleted larvae (Fig. 4q–s and Supplementary Fig. 3j, k ). Dilp6 induces Serrate via InR in blood progenitors We screened for increased expression of RNAs encoding neurosecretory peptides upon loss of CO 2 SN activity. Only one positive candidate, the Drosophila Insulin-like peptide-6 ( dilp6 ), is normally low in the fat body during larval stages [30] and is specifically upregulated in this organ when the CO 2 SN is mutated (Fig. 5a–d and Supplementary Fig. 4 a-d). While dilp6 is additionally expressed in glia [31] , we found that overexpression in the fat body, but not in glia, has an effect on CC number (Fig. 5e and Supplementary Fig. 4 e-g). Similarly, the CC phenotype due to reduced CO 2 SN activity is efficiently rescued when dilp6 is specifically blocked in the fat body or in the dilp6 41 mutant, but not when dilp6-RNAi is expressed in glial cells (Fig. 5f, g and Supplementary Fig. 4 h-k). Fig. 5 CO 2 SN/HypSNs systemically control Dilp6 and Serrate. e – g indicate the number of CCs in a single lymph gland lobe. Scale bar: 20μm; except in a, b : 50μm. n.s: not significant ( p > 0.01). * p < 0.01; ** p < 0.001; *** p < 0.0001. Error bars in c – d and h – l : standard deviation. Bars in graph e – g , x : the median. CO 2 SN inhibited conditions: –CO 2 R with shaded yellow in f, j–l . Soda-lime generated low CO 2 conditions: shaded blue in d , g . a–d Dilp6 secreted from the fat body is the second systemic signal. dilp6 is expressed upon loss of CO 2 SN activity ( Gr63a-LexA, LexAop-Shi ts1 ; Dilp6-gal4, UAS-GFP ) in the fat body (Dilp6, green) ( a , b , d ), but not the brain or blood ( c ). e–l dilp6 is necessary and sufficient in extra CC formation. Overexpression of dilp6 in the fat body is sufficient to induce CC differentiation ( ppl-gal4; UAS-dilp6 ) ( e ). Loss of dilp6 in the fat body reverts CCs in the CO 2 SN mutant background to wild-type numbers ( Gr63a-LexA, LexAop-Shi ts1 ; ppl-gal4, UAS-dilp6 RNAi ) ( f ). This is also seen under soda-lime treatment conditions ( ppl-gal4; UAS-dilp6 RNAi ) ( g ). Expression of either upd3 ( h ) or sima ( i ) in the brain is sufficient to enhance dilp6 expression in the fat body ( Elav-gal4; UAS-upd3 or Elav-gal4; UAS-sima ). Increased expression of dilp6 is disrupted by: silencing HypSNs ( Gr63a-LexA, LexAop-Shi ts1 ; Gyc89da-gal4, UAS-Shi ts1 ) ( j ), by sima RNA i in HypSNs ( Gr63a-LexA, LexAop-Shi ts1 ; Gyc89da-gal4, UAS-sima RNAi ) ( j ), upon inhibition of neuronal upd3 ( Gr63a-LexA, LexAop-Shi ts1 ; Elav-gal4, UAS-upd3 RNAi ) ( k ), or when dome RNAi is expressed in the fat body ( Gr63a-LexA, LexAop-Shi ts1 ; ppl-gal4, UAS-dome RNAi ) ( l ). m–x Insulin receptor (InR) activation by Dilp6 increases Serrate expression. pAKT (pAKT, red) ( m–n ) and p4EBP (p4EBP, red) ( o–p ) are upregulated in the lymph gland upon CO 2 SN inhibition ( Gr63a-gal4; UAS-Gr21a RNAi ). Compared with wild type ( q ), Serrate expression is substantially enhanced when CO 2 SN activity is lost ( Gr63a-gal4; UAS-hid,rpr ) (Serrate, red) ( r ). Neuronal expression of either sima ( Elav-gal4; UAS-sima ) ( s ) or upd3 ( Elav-gal4; UAS-upd3 ) ( t ), is sufficient to enhance Serrate protein expression. This phenotype is also seen when dilp6 is overexpressed in the fat body ( ppl-gal4; UAS-dilp6 ) ( u ). Su(H)-LacZ is activated in cells that receive active Notch signal. The number of such cells increases when CO 2 SN activity is attenuated ( Gr63a-gal4, Su(H)-LacZ; UAS-hid,rpr ) ( Su(H)-LacZ , red) ( v–w ). Quantitation is shown in x Full size image Overexpression of sima or upd3 in the brain raises fat body levels of dilp6 (Fig. 5h, i ). Increased dilp6 in a CO 2 SN activity-depleted background is suppressed: upon concurrent inhibition of HypSNs, with attenuation of brain sima or upd3 , or when dome-RNAi is expressed in the fat body (Fig. 5 j-l). A different insulin related peptide, Dilp2, functions in hematopoiesis, but not directly in CC formation [14] , [32] and no previously known role in hematopoiesis was identified for Dilp6. Both Dilps function by binding to the insulin receptor (InR), which is known to promote differentiation of CCs [16] , [32] . In CO 2 SN activity-depleted larvae, we detect high pAKT and p4EBP, direct phosphorylation targets of the InR pathway in the lymph gland (Fig. 5m–p and Supplementary Fig. 4 l-q). This is also seen when dilp6 is overexpressed in the fat body (Supplementary Fig. 4 r, s). We hypothesize that altered gaseous signaling leads to systemic secretion of Dilp6 from the fat body that activates InR pathway [30] , [31] , [33] . A hallmark of CC fate specification is the interaction between the ligand Serrate, expressed in internal signaling centers within the lymph gland, with its receptor Notch, present in neighboring cells [27] , [34] , [35] . Wild-type lymph glands from mid-second instar larvae exhibit low Serrate protein expression at the edge where differentiation is initiated (Fig. 5q ). Reduced CO 2 SN activity has a pronounced effect on membrane Serrate expression as this protein is detected in more cells at a much higher level when compared with wild type (Fig. 5r and Supplementary Fig. 4 t-v). Increased Serrate is also seen upon sima or upd3 overexpression in the brain, or when dilp6 is driven in the fat body (Fig. 5s–u ). We also detect an increase in number of cells in which Notch is active, but there is no change in the activation level per cell (Fig. 5v–x ). We conclude that the cascade leading up to InR increases Serrate expression, which in turn activates the Notch pathway in an increased number of cells causing them to take on CC fates. CC differentiation controlled by altered environmental gases A model summarizing the results presented in this study is shown in Fig. 6a . Environmental CO 2 activates its receptor Gr21a/Gr63a expressed on the CO 2 SN, while environmental levels of O 2 repress HypSNs. This occurs at the level of sensory neurons, and the information is relayed to higher brain centers. Genetic data support communication between these sensory neurons in the suboesophageal ganglion (SEG) and accumulation of Sima in a different set of HypSNs within a small number of VNC neurons. The neuronal circuits between the SEG, VNC and higher brain centers have not been mapped yet. However, it is clear that Sima enhances upd3 expression in the brain and that secretion of this cytokine activates the JAK/STAT pathway in the fat body and this results in Dilp6 expression and secretion into the hemolymph. The resulting Dilp6/InR signal within the lymph gland causes an increase in the level and number of cells that express Serrate. As is well known from the published literature, the Serrate–Notch interaction is critical in determining CC fate and number within the lymph gland [19] , [26] . The interorgan communication system identified in this study allows the monitoring of ambient gas levels in the environment and through their integration, allows any chronic imbalance of respiratory gases for the purpose of proper stress response and the maintenance of immune homeostasis. Fig. 6 Environmental alterations support results of genetic manipulations. b–d indicate the number of CCs in a single lymph gland lobe. Scale bar: 20μm. n.s: not significant ( p > 0.01). * p < 0.01; ** p < 0.001; *** p < 0.0001. Error bars in i – q : standard deviation. Bars in graph b – d , h : the median. Soda-lime generated low CO 2 conditions: blue; hypoxic (10% O 2 ) conditions: green; hyperoxic (40% O 2 ) conditions: pink. a A model summarizing the systemic response events. b–d Physiological relevance probed by altering environmental gases. Environmental CO 2 is scavenged by soda-lime. Hypoxic (<10% O 2 ) or hyperoxic (>40% O 2 ) conditions are achieved in hypoxia chambers. Elimination of CO 2 using soda-lime significantly increases the number of CCs in the lymph gland, and this response is further aggravated by the concurrent loss of CO 2 SN ( Gr63a-gal4; UAS-Gr21a RNAi ) ( b ). Hypoxia increases CC number, but this phenotype cannot be further enhanced by low CO 2 SN activity ( Gr63a-gal4; UAS-Gr21a RNAi ) ( c ). Hyperoxia on its own significantly suppresses CC development, and also efficiently rescues the low CO 2 SN-induced CC differentiation to normal levels ( d ). e–q Phenotypic parallels between decreased levels of ambient CO 2 and O 2 . In addition to low CO 2 SN activity induced by genetic manipulation (Fig. 3a–c) , soda-lime treatment accumulates Sima protein expression in a specific subset of VNC neurons ( e , f ). Similar accumulation of Sima is observed by rearing larvae in hypoxic conditions ( g ). Quantitation shown in h . Both hypoxia and soda-lime treatments enhance upd3 in the brain ( i–j ), Socs36e and dilp6 transcript levels in the fat body ( l–m , o–p ). This expression is not observed in hyperoxia treatment ( k , n , q ) Full size image A unique feature of this model is the integration of CO 2 and O 2 sensation to achieve a common blood phenotype. For the results to be physiologically relevant, alteration of environmental gaseous ligands should phenocopy the effects of genetic manipulations. The normal atmosphere contains approximately 0.04% of CO 2 with additional CO 2 released from fermenting food sources. Environmental CO 2 is scavenged in larval culture vials with the use of a mixture of bases, “soda-lime” (see Supplementary Fig. 1c and Methods). The soda-lime method scavenges atmospheric CO 2 to very low levels without altering development, while hypoxia chambers can create controlled hypoxia, hyperoxia, or hypercapnia environments. Most importantly, exposure of wild-type larvae to either soda-lime or to hypoxia increases CC numbers (Fig. 6b, c and Supplementary Fig. 5a, b compare with the genetic manipulations in Fig. 1i ). Lowering CO 2 SN activity does not further enhance the hypoxia phenotype (Fig. 6c and Supplementary Fig. 5c ). On its own, hyperoxia decreases CC numbers compared to wild type and also suppresses the low CO 2 SN-activity phenotype (Fig. 6d and Supplementary Fig. 5d, e compare Fig. 2d, i ), whereas hypercapnia does not alter the CC formation (Supplementary Fig. 5f ). Finally, soda-lime and hypoxia both: increase nuclear Sima in neurons (Fig. 6 e-h compare Fig. 3 a-f), and increase upd3 in the brain (Fig. 6i–k compare Fig. 4a, b ), and Socs36e (Fig. 6l–n compare Fig. 4n, p ) and dilp6 in the fat body (Fig. 6o–q compare Fig. 5c, j ). These results demonstrate that the CC phenotypes can be triggered by imbalances in respiratory gases in wild-type animals, establishing a physiological relevance for our observations. A wild-type number of CCs is generated through local developmental signals independent of sensory input [27] , [34] , [35] . The multi-organ and multi-pathway cascade described here represents a stress signal activated upon alteration in respiratory gases over the developmental time period. Such sustained variations in gaseous components are likely to be experienced fairly often during larval development. During the time period over which hematopoiesis is at its peak within the lymph gland, larvae experience hypoxic conditions buried into the food that they forage through. Decomposition and yeast (a primary food source) cause variations in CO 2 levels. Toward the end of the hematopoietic developmental period, larvae spend extended periods of time in a very different environment awaiting pupariation. Finally, molting is associated with the shedding of the cuticular intima and degeneration of tracheoles that lack these inner linings [36] . As the tracheal tube is filled with fluid and devoid of gases at this stage, we speculate that this process is also likely to alter oxygen tension in the hemolymph. In past studies, CCs have been associated with hypoxia and hypoxic stress as well as innate immune response [23] , [27] , [37] . How increased numbers of these cells will mitigate the effects of gaseous imbalance will require detailed analysis in the future. However, in order to determine whether the presence of CCs provides a benefit to the whole animal, we generated flies in which the final step in the cascade, Serrate, is eliminated in cells from which CCs are derived during larval development. We then tested the emerging adults for sensitivity to hypoxia and found that these flies fully paralyze in a hypoxia chamber much more readily than genetically matched control flies (Supplementary Fig. 5 g, h; the p -value is <0.0001). Thus, in addition to their other functions, CCs provide general protection against hypoxia to the animal. For myeloid progenitors, which are sentinels for stress and infection, we consistently find that stress signals feed into developmental pathways, in this case Serrate–Notch signaling, to enhance the homeostatic response to a level more appropriate for rapid immune and stress response [9] , [38] . To determine if loss of gaseous sensation is linked to innate immunity, we tested levels of antimicrobial peptides in animals lacking CO 2 SN. 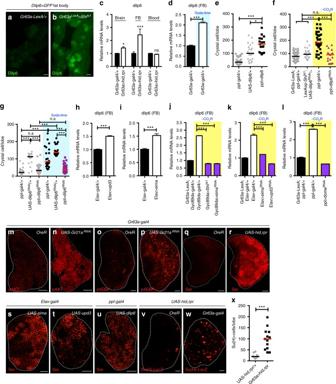Fig. 5 CO2SN/HypSNs systemically control Dilp6 and Serrate.e–gindicate the number of CCs in a single lymph gland lobe. Scale bar: 20μm; except ina, b: 50μm. n.s: not significant (p> 0.01). *p< 0.01; **p< 0.001; ***p< 0.0001. Error bars inc–dandh–l: standard deviation. Bars in graphe–g,x: the median. CO2SN inhibited conditions: –CO2R with shaded yellow inf, j–l. Soda-lime generated low CO2conditions: shaded blue ind,g.a–dDilp6 secreted from the fat body is the second systemic signal.dilp6is expressed upon loss of CO2SN activity (Gr63a-LexA, LexAop-Shits1; Dilp6-gal4, UAS-GFP) in the fat body (Dilp6, green) (a,b,d), but not the brain or blood (c).e–ldilp6is necessary and sufficient in extra CC formation. Overexpression ofdilp6in the fat body is sufficient to induce CC differentiation (ppl-gal4; UAS-dilp6) (e). Loss ofdilp6in the fat body reverts CCs in the CO2SN mutant background to wild-type numbers (Gr63a-LexA, LexAop-Shits1;ppl-gal4, UAS-dilp6RNAi) (f). This is also seen under soda-lime treatment conditions (ppl-gal4; UAS-dilp6RNAi) (g). Expression of eitherupd3(h) orsima(i) in the brain is sufficient to enhancedilp6expression in the fat body (Elav-gal4; UAS-upd3orElav-gal4; UAS-sima). Increased expression ofdilp6is disrupted by: silencing HypSNs (Gr63a-LexA, LexAop-Shits1;Gyc89da-gal4, UAS-Shits1) (j), bysimaRNAiin HypSNs (Gr63a-LexA, LexAop-Shits1;Gyc89da-gal4, UAS-simaRNAi) (j), upon inhibition of neuronalupd3(Gr63a-LexA, LexAop-Shits1;Elav-gal4, UAS-upd3RNAi) (k), or whendomeRNAiis expressed in the fat body (Gr63a-LexA, LexAop-Shits1;ppl-gal4, UAS-domeRNAi) (l).m–xInsulin receptor (InR) activation by Dilp6 increases Serrate expression. pAKT (pAKT, red) (m–n) and p4EBP (p4EBP, red) (o–p) are upregulated in the lymph gland upon CO2SN inhibition (Gr63a-gal4; UAS-Gr21aRNAi). Compared with wild type (q), Serrate expression is substantially enhanced when CO2SN activity is lost (Gr63a-gal4; UAS-hid,rpr) (Serrate, red) (r). Neuronal expression of eithersima(Elav-gal4; UAS-sima) (s) orupd3(Elav-gal4; UAS-upd3) (t), is sufficient to enhance Serrate protein expression. This phenotype is also seen whendilp6is overexpressed in the fat body (ppl-gal4; UAS-dilp6) (u).Su(H)-LacZis activated in cells that receive active Notch signal. The number of such cells increases when CO2SN activity is attenuated (Gr63a-gal4, Su(H)-LacZ; UAS-hid,rpr) (Su(H)-LacZ, red) (v–w). Quantitation is shown inx 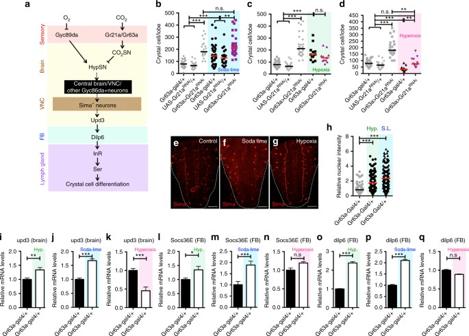Fig. 6 Environmental alterations support results of genetic manipulations.b–dindicate the number of CCs in a single lymph gland lobe. Scale bar: 20μm. n.s: not significant (p> 0.01). *p< 0.01; **p< 0.001; ***p< 0.0001. Error bars ini–q: standard deviation. Bars in graphb–d,h: the median. Soda-lime generated low CO2conditions: blue; hypoxic (10% O2) conditions: green; hyperoxic (40% O2) conditions: pink.aA model summarizing the systemic response events.b–dPhysiological relevance probed by altering environmental gases. Environmental CO2is scavenged by soda-lime. Hypoxic (<10% O2) or hyperoxic (>40% O2) conditions are achieved in hypoxia chambers. Elimination of CO2using soda-lime significantly increases the number of CCs in the lymph gland, and this response is further aggravated by the concurrent loss of CO2SN (Gr63a-gal4; UAS-Gr21aRNAi) (b). Hypoxia increases CC number, but this phenotype cannot be further enhanced by low CO2SN activity (Gr63a-gal4; UAS-Gr21aRNAi) (c). Hyperoxia on its own significantly suppresses CC development, and also efficiently rescues the low CO2SN-induced CC differentiation to normal levels (d).e–qPhenotypic parallels between decreased levels of ambient CO2and O2. In addition to low CO2SN activity induced by genetic manipulation (Fig.3a–c), soda-lime treatment accumulates Sima protein expression in a specific subset of VNC neurons (e,f). Similar accumulation of Sima is observed by rearing larvae in hypoxic conditions (g). Quantitation shown inh. Both hypoxia and soda-lime treatments enhanceupd3in the brain (i–j),Socs36eanddilp6transcript levels in the fat body (l–m,o–p). This expression is not observed in hyperoxia treatment (k,n,q) Indeed, loss of CO 2 sensation is associated with a four to six-fold increase in the transcription of Drosomycin and a four-fold increase for Drosocin (Supplementary Fig. 5i ). However, the significance of this response by the blood cells in the absence of any microbial infection is not clear. We attribute this global and preemptive augmentation of the innate immune system to the increased concentrations of cytokines such as Upd3 and Dilp6 that result from long-term loss of gaseous sensation. Additional physiological effects such as altered lifespan in Drosophila [39] and innate immune response in C. elegans [40] , [41] have been associated with CO 2 and O 2 sensation. Together, these studies allow us to infer that O 2 and CO 2 chemosensation has a conserved role in animal physiology and immunity. Although the mechanistic details are not yet deciphered, it seems clear that this conservation extends to mammalian species including humans. Several studies suggest a crosstalk between CO 2 and O 2 in mammals [42] and establish an influence of gaseous sensation on the hematopoietic system [43] , [44] . The ventral surface of the mammalian medulla oblongata senses CO 2 [45] and responds to O 2 sensing by the carotid chemoreceptor neurons [46] , [47] . Chemosensation and immunity are closely linked and each is evolutionarily conserved at a mechanistic level. Whether a multi-organ cascade involving multiple cytokines similar to that described in this study links gaseous signaling to myeloid cell function and development in humans will be attractive to investigate. Drosophila stocks and genetics The following Drosophila stocks were used in this study: Gr63a-gal4 (BL9942), Gr21a-gal4 (BL24147), Gyc89da-gal4 and Gyc89da-GFP (D. Morton), Elav-gal4 (BL8765), ppl-gal4 (BL58768), HHLT-gal4 (C. Evans), Upd3-gal4 (H. Agaisse), Repo-gal4 (BL7415), Dilp6-gal4 (A. Brand), HmlΔ-gal4 (S. Sinenko), Hml-dsRed; Dome-Meso-GFP (U. Banerjee) , Gr21a RNAi (BL31281 and VDRC104122), dilp6 RNAi (BL33684 and VDRC102465), upd3 RNAi (VDRC106869), sima RNAi (VDRC106187), dome RNAi (VDRC19717), Gad1 RNAi (BL51794), GBR1 RNAi (VDRC101440), GBR2 RNAi (BL50608), Serrate RNAi (VDRC27172), UAS-sima (BL9582), UAS-dilp6 (E. Hafen), UAS-upd3 (B. Lemaitre), UAS-hid, rpr (Nambu JR), UAS-Shi ts1 (T. Kitamoto), UAS-syb::GRASP (BL64315), UAS-CD4::GRASP (BL58755), UAS-GTrace (C. Evans), UAS-NaChBac (BL9469), UAS-mCD8GFP (BL5137), UAS-DenMark (BL33063), Elav-gal80 (Y.N. Jan), LexAop-Shi ts1 (G. Rubin), 13XLexAop2-6XmCherry-HA (BL52271), 12xSu(H)-LacZ (S. Artavanis-Tsakonas), Gr63a 1 (BL9941), Df[Gr21a] (DGRC150003), dilp6 41 (BL30885), upd2Δupd3Δ (BL55729), upd3Δ( BL55728). Generation of Gr63a-LexA , Gyc89da-LexA and Lz-LexA flies: Gr63a enhancer [4] , Gyc89da enhancer [20] or Lz enhancer (Forward primer sequence:GGGATTAGGCAGTGTTCCC, Reverse primer sequence:GTACCAATCGCTCCATCCAC) was amplified from fly genomic DNA and ligated into the TOPO-TA vector (Invitrogen) for Gateway cloning. Each entry vector was ligated into the pBPnlsLexA::p65Uw (Addgene 26230) destination vector using the LR ligase (Invitrogen). Transgenic flies were generated by BestGene Inc. All fly stocks were maintained at 18 °C. Unless indicated, crossed flies were maintained at 29 °C with dextrose-cornmeal based conventional food for maximum Gal4-UAS/LexA-LexAoP expression. Experiments with soda-lime/hypoxia/hyperoxia/hypercapnia and synchronization [15] of larvae were performed at 25 °C. Gyc89da-gal4 crossed with UAS-sima flies were maintained at 18 °C until reaching the mid-second instar (approximately 5 days) and shifted to 25 °C. 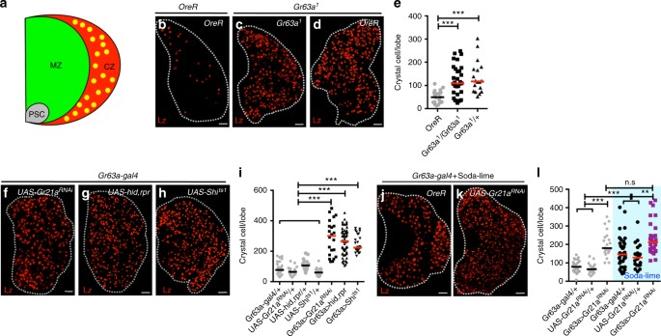Elav-gal4 crossed with UAS-sima or UAS-upd3 , or Gyc89da-gal4 crossed with UAS-NaChBac was maintained at 25°C. These above four genotypes show a drowning or lethal phenotype at 29 °C. Gr63a 1 mutants were back-crossed more than 50 generations. Gyc89da-gal4 or Dilp6-gal4 was recombined with UAS-mCD8GFP ; Gyc89da-LexA , or Lz-LexA was recombined with 13xLexAoP2-6XmCherry-HA . Fig. 1 CO2chemosensation controls the differentiation of crystal cells. Graphs indicate the number of crystal cells (CC) per lymph gland lobe. Bars in graphs: the median. n.s: not significant (p> 0.01). *p< 0.01; **p< 0.001; ***p< 0.0001. Scale Bar: 20μm. White dotted lines: lymph glands. Statistical results and genotypes are indicated in Supplementary Table3.aA schematic representation of the primary lobe of the hematopoietic organ, the larval lymph gland. Undifferentiated blood progenitors reside in the inner core, termed the medullary zone (MZ), and give rise to mature blood cell lineages including crystal cells (CC, marked in yellow) that occupy a region termed the cortical zone (CZ). The posterior signaling center (PSC) secretes multiple factors to maintain the progenitors. Only the features relevant to this study are shown.b–lLoss of CO2SN activity causes increased CC number. Wild-type third-instar larvae express fewer than 100-CCs per primary lymph gland lobe (CCs are marked in red, Lz) (b) Both homozygous (Gr63a1/Gr63a1) (c) and heterozygous (Gr63a1/+) mutants (d) ofGr63a, the gene encoding the chemoreceptor for CO2sensing, exhibit increased numbers of CCs. Quantitation of CC numbers shown in (e).Gr21aencodes the second subunit of the CO2chemoreceptor that functions withGr63a. Knockdown ofGr21afunction (Gr63a-gal4; UAS-Gr21aRNAi) (f), or genetic ablation of the CO2receptor neuron by expression of pro-apoptotic genes,hidandrpr(Gr63a-gal4; UAS-hid,rpr) (g) or attenuation of synaptic transmission by expression of a temperature-sensitive form of the dynamin-like protein Shibire (Gr63a-gal4; UAS-Shits1) (h), each causes a significant increase in the number of CCs. This phenotype is not observed inGal4- orUAS-controls alone. Quantitation is shown ini. Absorption of ambient CO2in larval culture vial with the use of soda-lime, a mixture of bases that eliminates gaseous CO2(see Methods for detail), mimics the CO2SN mutant phenotype (j). This phenotype is enhanced by a simultaneous knockdown ofGr21ain the CO2SN (Gr63a-gal4; UAS-Gr21aRNAi) (k). Quantitation shown inl. The blue shading in panels (l) represents soda-lime-induced low environmental CO2condition Efficiencies of RNA i lines used in this study are indicated in Supplementary Table 1 . Soda-lime, CO 2 , and O 2 control experiments For the soda-lime treatment: the soda-lime (Sigma 72073) experiment was designed based on the previous study [48] . To avoid crowding, eight females and six male flies were crossed for all experiments and vials were shifted to new vials every day. Twenty soda-lime particles were wrapped and sealed with gauze (referred to as a soda-lime pocket). This soda-lime pocket was attached 5 mm above the food to diminish metabolic CO 2 emitted from larvae. To eliminate atmospheric CO 2 , a 1000 μL pipette tip containing fifteen loosely-packed particles of soda-lime was inserted into a vial sealed with parafilm (Supplementary Fig. 1c ). Putting more than twenty soda-lime particles in the pipette tip inhibits air flow and putting the pocket inside the food negatively affected larval growth. With this number of soda-lime particles, there was no developmental influence on larvae. Experiments were independently repeated at least three times. For O 2 and CO 2 modulation experiments: hypoxia, hyperoxia and hypercapnia experiments were done in a hypoxia chamber (Modular Incubator Chamber MIC-101, Billups-Rothenberg.Inc or ProOX C21, BioSpherix). 10% (±0.5%) O 2 was used for hypoxia experiments, 40% (±0.5%) O 2 for hyperoxia, 13% (±0.5%) CO 2 for hypercapnia. Drosophila larvae were synchronized and cultured in normoxic conditions until 72 h after egg laying, and shifted to either hypoxic or hyperoxic condition. After rearing animals for 48 h in the chamber, wandering third-instar larvae were dissected immediately. For hypercapnia, the first-instar larvae were synchronized and shifted to the chamber, and dissected when they reached the wandering third-instar. Hypoxia/hyperoxia/hypercapnia and soda-lime experiments were done at 25 °C. Immunohistochemistry Lymph glands were dissected and stained as previously described [8] . Following primary antibodies were used in this study: αLz (DSHB, 1:10), αSima [49] (1:100), αβgal (Promega, 1:1000), αnc82 (DSHB, 1:10), αAntp (DSHB, 1:10), αp4EBP (Cell signaling, 2855 S, 1:100), αpAKT (Cell signaling, 4060 S, 1:100) and αSerrate (K. Irvine, 1:1000). Cy3-, FITC- or Alexa Fluor 647-conjugated secondary antibody (Jackson Laboratory) was used for staining. Alexa Flour 594 Phalloidin (Thermo Fisher, A12381) was used for F-actin staining. All samples were mounted in VectaShield (Vector Laboratory) and imaged by Zeiss Axiocam 503, Nikon C2 Si-plus or Zeiss LSM880 Airyscan confocal microscopy. For αSerrate staining, a pre-absorption step was essential for clear lymph gland staining. To do so, a 1:100 concentration (2% sodium azide) of antibody was incubated together with nine fixed larval cuticles overnight at 4 °C. Lymph glands were dissected at 72 h AEL and fixed in 3.7% formaldehyde for 25 min at room temperature. After fixation, lymph glands were washed 3 times (10 min each) nutating in 0.1% Tween20 in 1 × PBS and blocked in 1% BSA/0.1% Tween20 in 1xPBS for 30 min on a table-top shaker. Lymph glands were incubated overnight in αSerrate primary antibody (used at a final concentration of 1:1000) at 4 °C. Lymph glands were washed 3 times (10 min each) nutating in 0.1% Triton-X in 1xPBS and then incubated in Rat secondary antibody with 1% BSA/0.1% Triton-X in 1xPBS for 3 h at room temperature. 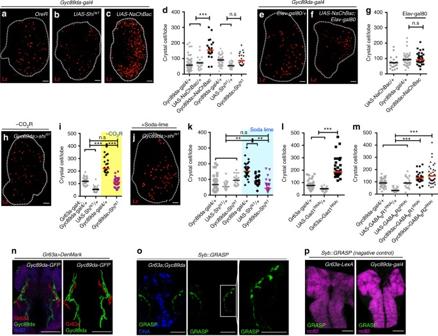After washing 3 times (10 min each) with 0.1% Triton-X in 1xPBS, samples were mounted in Vectashield with DAPI and imaged as described above. Quantitative real-time PCR analysis At least 20 larval organs (at least 100 for the lymph gland) were dissected to extract RNA. cDNA was synthesized with qPCR-RT kit (TOYOBO). qRT-PCR was performed by comparative C T method using SYBR Green Realtime PCR Master Mix (TOYOBO) and a StepOne-Plus Real-Time PCR detection thermal cycler (Applied Biosystems). Fig. 2 CO2SN forms inhibitory synapses with HypSN. Graphs indicate the number of crystal cells (CC) per lymph gland lobe. Bars in graphs: the median. n.s: not significant (p> 0.01). *p< 0.01; **p< 0.001; ***p< 0.0001. Scale Bar: 20μm, unless otherwise indicated. White dotted lines: lymph glands. CO2SN inhibited conditions: –CO2R with shaded yellow ini, and Soda-lime generated low CO2: shaded blue inkfor clarity.a–gConstitutive activation of HypSNs induces CC differentiation. Control animals (Gyc89da-gal4/+) have an average of 70-90 CCs (a). Inactivation of HypSNs (Gyc89da-gal4; UAS-Shits1) does not alter CC number (b). Constitutive activation of HypSNs by expressing the bacterial sodium channel, NaChBac (Gyc89da-gal4; UAS-NaChBac) results in increased CC differentiation (c). Quantitation is shown ind. When the expression of NaChBac is specifically blocked in neurons (Gyc89da-gal4, Elav-gal80; UAS-NaChBac) the average CC number is unchanged (f) from that in control (e). Quantitation shown ing. h–kHypSNs function downstream of CO2SN. As shown in (Fig.1h), CO2SN inhibition increases CC number (Gr63a-gal4; UAS-Shits1). This phenotype reverts to wild type when HypSNs are also inhibited (Gr63a-gal4; Gyc89da-gal4, UAS-Shits1) (h). Quantitation shown ini. Soda-lime-mediated CC phenotype is also alleviated by inhibition of HypSNs (low atmospheric CO2+Gyc89da-gal4; UAS-Shits1) (j). Quantitation shown ink.l–mGABA-mediated inhibition of HypSNs by CO2SN. Knockdown ofGad1in the CO2SN (Gr63a-gal4; UAS-Gad1RNAi) enhances differentiation of CCs (l). Similarly, loss of eitherGABABR1orGABABR2in HypSNs (Gyc89da-gal4; UAS-GABABR1RNAiorGyc89da-gal4; UAS-GABABR2RNAi) also leads to increased CC differentiation (m).n–oPhysical proximity and overlap of CO2SN and HypSNs in the SEG. Projections of the CO2SN adjoining HypSNs at the level of the SEG shows significant co-localization: CO2SN in red and HypSN in green (Gr63a-gal4; UAS-DenMark; Gyc89da-GFP). Rendered image of the co-localization data shown in right panel (n). Syb::GRASP expression of the CO2SN and HypSNs in the SEG (o). Syb::GRASP signal resulting from points of contact is shown in green (Magnified images in the following panels) (o). pNegative control experiments for the Syb::GRASP data shown ino.Gr63a-LexAalone (Gr63a-LexA; UAS-CD4-spGFP11, LexAop-nSyb-spGFP1-10) orGyc89da-gal4alone (Gyc89da-gal4; UAS-CD4-spGFP11, LexAop-nSyb-spGFP1-10) does not give rise to a GRASP signal. Scale bar: 50μm Specific primers used for qRT-PCR are described in Supplementary Table 2 . Quantification of samples CCs were quantified and analyzed by ImageJ (plug in: 3D object counter) or Imaris (Bitplane). CCs in individual primary lobes were counted for this study. Whole Z-stacks were compressed and analyzed for the quantification and figure presentation. Other stainings including pAKT, p4EBP or Serrate are shown in a single middle Z-stack slice. For CCs in circulation, Lz-LexA LexAop-mCherry positive blood cells in a larva were counted after bleeding. Prior to bleeding, animals were vortexed for 2 min to detach sessile population. Statistical significance of the CC phenotype was analyzed by Wilcoxon rank sum test after determining normality with the use of SPSS. Given natural variability of the number of CCs, we considered samples are significantly different only when * p < 0.01. Statistical results and genotypes are indicated in Supplementary Table 3 . Relative nuclear Sima intensity was analyzed with the use of IMARIS software. Amongst Sima immunoreactivity shown in the brain, we only selected high Sima + cells to avoid background expressions, and of which nuclear intensity was measured and calculated. Relative intensity of mutants compared to wild type was presented in figures. Hypoxia tolerance experiment Three-day-old male flies were used for hypoxia tolerance experiments. 15 flies were placed in one empty vial and conditioned for 2 h before transferring to 1% oxygen-containing hypoxia chamber. Fly movement was recorded for 1 h. 1 point was given when any fly from one vial shows a movement in 5 s; therefore, 12 point per 1 min for maximum. Flies were never placed in hypoxic condition before this experiment. Behavior assay was repeated more than three times with biologically independent samples. Data availability All data generated during and/or analyzed during the current study are included in this published article and its supplementary information files.